Delayed bactericidal response ofMycobacterium tuberculosisto bedaquiline involves remodelling of bacterial metabolism Bedaquiline (BDQ), an ATP synthase inhibitor, is the first drug to be approved for treatment of multidrug-resistant tuberculosis in decades. Though BDQ has shown excellent efficacy in clinical trials, its early bactericidal activity during the first week of chemotherapy is minimal. Here, using microfluidic devices and time-lapse microscopy of Mycobacterium tuberculosis , we confirm the absence of significant bacteriolytic activity during the first 3–4 days of exposure to BDQ. BDQ-induced inhibition of ATP synthesis leads to bacteriostasis within hours after drug addition. Transcriptional and proteomic analyses reveal that M. tuberculosis responds to BDQ by induction of the dormancy regulon and activation of ATP-generating pathways, thereby maintaining bacterial viability during initial drug exposure. BDQ-induced bacterial killing is significantly enhanced when the mycobacteria are grown on non-fermentable energy sources such as lipids (impeding ATP synthesis via glycolysis). Our results show that BDQ exposure triggers a metabolic remodelling in mycobacteria, thereby enabling transient bacterial survival. Tuberculosis (TB) still claims more human lives each year than any other bacterial infection [1] . The latest report from the World Health Organization revealed signs of progress against drug-susceptible TB; however, the incidence rates of multidrug-resistant TB (MDR-TB) have sharply increased, thereby threatening global TB control programs [1] , [2] . Recent clinical data from two controlled phase 2 trials have revealed the efficacy of a novel anti-TB drug, bedaquiline (BDQ, marketed as Sirturo), in treatment of MDR-TB [3] , [4] . On the basis of the surrogate end point of time-to-sputum culture conversion, BDQ was granted accelerated approval by the US Food & Drug Administration for the treatment of pulmonary MDR-TB as part of combination therapy in adults [5] , [6] . This marks the first regulatory approval of an anti-TB drug since the introduction of rifampin in 1971. BDQ is a first-in-class ATP synthase inhibitor, displaying high selectivity for mycobacterial ATP synthase [7] , [8] , [9] , thus highlighting the key role of energy metabolism as a novel drug target pathway in mycobacteria [10] , [11] , [12] . BDQ exhibited potent bactericidal activity both in mouse models of TB infection [7] , and also when given for either 2 or 6 months in combination with a background regimen in MDR-TB patients [3] , [4] . However, its bactericidal activity in extended early bactericidal activity (eBA) studies showed a delayed onset, with the decline in bacterial sputum counts observed only from day 4–6 onwards [13] , [14] , [15] . This delay in onset of bactericidal activity is not simply due to the inability of the drug to reach steady state levels in patients, as a similar delay was seen in in vitro studies [7] , [16] . Similar to BDQ, the front-line anti-TB drug pyrazinamide also displays almost no bactericidal activity during the first 2–4 days of treatment, but nonetheless it kills consistently thereafter [12] . However, pyrazinamide was developed in 1950s in a different regulatory environment. Today, eBA is used for establishing a quick clinical proof of concept, and unfavourable eBA is regarded as an impediment for drug development. eBA studies are traditionally carried out over a period of 2–7 days, consequently eBA may underestimate the potency of drugs with a delayed onset of bactericidal activity. As such, insight into microbiological and molecular factors underlying the delayed onset of bactericidal activity by BDQ may provide valuable information for the design and interpretation of eBA studies on new drug candidates. In the current report, we aim at understanding the reason for the delayed onset of killing by BDQ. We investigate individual cells of M. tuberculosis in microfluidic devices and show the absence of bacteriolysis in mycobacteria during the initial days of BDQ treatment. We employ multiple biochemical and molecular approaches and elucidate temporal changes in bacterial metabolic pathways upon BDQ exposure. We show bacteria tend to minimize the consumption of cellular ATP and at same time enhance the capacity of ATP-generating pathways, which contributes to maintaining bacterial viability in spite of antibiotic stress. We also investigate the impact of the employed energy source on mycobacterial susceptibility to BDQ and demonstrate that mycobacteria grown on lipids display enhanced BDQ mediated killing. These data reveal how metabolic remodeling upon drug exposure can enable transient bacterial survival. Our results also indicate that inhibitors of mycobacterial ATP synthesis may prove powerful drugs for eradicating mycobacteria growing in lipid-rich environments in the human host. This shows that non-fermentable energy sources can be explored for in vitro characterization of new molecules targeting mycobacterial energy pathways. Finally, these data highlight that drugs specifically targeting the mycobacterial respiratory chain components like ATP synthase or cytochrome bc1, may exhibit a delayed onset of bactericidal activity both in vitro as well as in clinical eBA type studies within TB patients. Delayed killing of M . tuberculosis by BDQ We correlated the killing activity of BDQ with its impact on cellular ATP levels, in particular during the initial days of drug exposure. We confirmed that BDQ was highly bactericidal on M. tuberculosis over a period of 18 days in vitro , leading to a drop of ~4 log 10 units in colony forming units (CFUs) by day 14 ( Fig. 1a ). However, during the first 2 days BDQ showed very little bactericidal activity, with <1 log 10 unit of killing observed by day 4, even at 300 × minimal inhibitory concentration (MIC) (MIC 99 of BDQ is 0.03 μg ml −1 ) [7] ( Fig. 1b ). Simultaneous measurements of bacterial ATP levels revealed a 1,000-fold drop in cellular ATP levels by day 9 at 300 × MIC ( Fig. 1c ). Nevertheless, during the first 2 days of BDQ exposure <10-fold drop in ATP levels was observed at 300 × MIC, with minimal changes at drug concentrations of 3 or 30 × MIC ( Fig. 1d ). As a control, isoniazid a potent inhibitor of cell envelope lipid biosynthesis had no effect on ATP levels, even at 300 × MIC ( Fig. 1c,d ). Moreover, a BDQ-resistant M. tuberculosis strain carrying point mutations in ATP synthase [7] did not show any decrease in ATP levels at all drug concentrations tested, demonstrating target specificity ( Fig. 1d , inset). ATP synthase is essential for growth in mycobacteria [17] , [18] and its inhibition by BDQ efficiently shuts down the function of this key metabolic enzyme. However, the decrease in ATP levels observed during the initial 2-day period of BDQ exposure did not sufficiently interfere with bacterial viability ( Fig. 1b,d ), suggesting that, at the population level, ATP levels need to be reduced by more than 1 log 10 unit before significant killing starts. Consistent with this result, previously it has been shown that dormant M. tuberculosis cultures are viable with ~10-fold lower ATP levels as compared with replicating bacteria, but are efficiently killed upon further ATP depletion [19] . 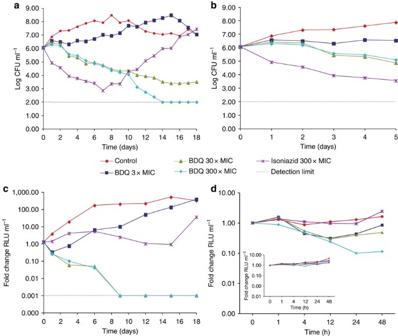Figure 1: Delayed killing ofM. tuberculosisby BDQ. (a) Kill kinetics of BDQ forM. tuberculosisover a period of 18 days and (b) initial 5 days of the BDQ kill kinetics. The bacteria were grown in liquid culture (Middlebrook 7H9 medium) in the presence of the indicated concentrations of BDQ or the front-line anti-TB drug isoniazid as a control. (c) Decrease of cellular ATP levels inM. tuberculosisduring 18 days of BDQ treatment. (d) Cellular ATP levels during the initial 48 h of BDQ treatment. Inset: cellular ATP levels in the BDQ-resistantM. tuberculosisstrain. ATP levels were determined using the bioluminescence method and are displayed as relative luminescence units (RLUs). Representative results from two experiments are shown. Figure 1: Delayed killing of M. tuberculosis by BDQ. ( a ) Kill kinetics of BDQ for M. tuberculosis over a period of 18 days and ( b ) initial 5 days of the BDQ kill kinetics. The bacteria were grown in liquid culture (Middlebrook 7H9 medium) in the presence of the indicated concentrations of BDQ or the front-line anti-TB drug isoniazid as a control. ( c ) Decrease of cellular ATP levels in M. tuberculosis during 18 days of BDQ treatment. ( d ) Cellular ATP levels during the initial 48 h of BDQ treatment. Inset: cellular ATP levels in the BDQ-resistant M. tuberculosis strain. ATP levels were determined using the bioluminescence method and are displayed as relative luminescence units (RLUs). Representative results from two experiments are shown. Full size image Single-cell analysis of the effect of BDQ on M. tuberculosis It is possible that the delayed onset of bacterial killing is due to the ability of the bacterial population or a subset of the population to continue growing and dividing using either stored ATP resources or by surviving on the depleted ATP levels. To address this issue, we studied the effect of BDQ on M. tuberculosis using time-lapse imaging of individual bacteria grown in microfluidic devices. In the presence of BDQ at 300 × MIC cell lysis was not observed until 3–4 days after drug addition ( Fig. 2a , Supplementary Movie 1 ), consistent with the lack of bactericidal activity observed in our in vitro kill kinetics assays. However, BDQ addition resulted in decrease of the bacterial growth rate within 12 h ( Fig. 2b ). Thus, using microscopy-based real-time visualization of BDQ action, we were able to establish that the delay in bactericidal activity seen with BDQ was not due to a heterogeneous response in the bacterial population. In fact, the entire population uniformly decreased their growth rate ( Fig. 2b , Supplementary Movie 1 ). Very few cell lysed during the first 100 h of BDQ exposure ( Supplementary Fig. 1a ). However, after this lag period a significant fraction of cells began to lyse ( Supplementary Fig. 1b ). This rate of cell lysis continued even after the drug washout (from day 17 to 24 ( Fig. 2a , Supplementary Fig. 1b )), with similar kinetics as during the drug exposure, suggesting strong post-antibiotic killing mediated by BDQ. As an end point assay we carried out propidium iodide staining to determine the fraction of intact cells with compromised cell membranes. Interestingly, we did not observe any regrowth after drug washout, even though a significant number of green fluorescent protein (GFP)-positive intact cells were found to be propidium iodide negative (34.8%) ( Supplementary Fig. 1b ), in line with a pronounced post-antibiotic effect. 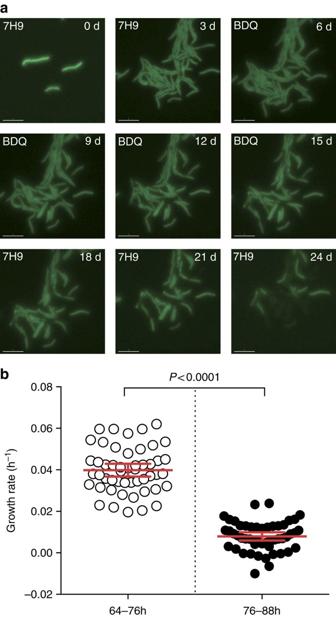Figure 2: Real-time single-cell analysis of effect of BDQ onM. tuberculosis. M. tuberculosisexpressing GFP was grown in a microfluidic device and imaged over a 24-day period at 1-h intervals. BDQ (300 × MIC) was added to the flow medium betweent=76–412 h (days 3–17). (a) Snapshot images of a representative microcolony imaged on the green channel are shown. Numbers (upper right) indicate days elapsed. Labels (upper left) indicate presence or absence of BDQ in the flow medium (7H9). Scale bar, 5 μm. (b) Single-cell growth rates were determined by measuring the areas of single cells (n=50) in the 12 h before BDQ exposure (64–76 h) and in the immediate 12 h after BDQ exposure (76–88 h) and fitting exponential curves to the data. Red lines represent the mean ± 95% confidence intervals. For comparison of growth rates,P-values were determined using the Kolmogorov–Smirnov non-parametric test. Figure 2: Real-time single-cell analysis of effect of BDQ on M. tuberculosis . M. tuberculosis expressing GFP was grown in a microfluidic device and imaged over a 24-day period at 1-h intervals. BDQ (300 × MIC) was added to the flow medium between t =76–412 h (days 3–17). ( a ) Snapshot images of a representative microcolony imaged on the green channel are shown. Numbers (upper right) indicate days elapsed. Labels (upper left) indicate presence or absence of BDQ in the flow medium (7H9). Scale bar, 5 μm. ( b ) Single-cell growth rates were determined by measuring the areas of single cells ( n =50) in the 12 h before BDQ exposure (64–76 h) and in the immediate 12 h after BDQ exposure (76–88 h) and fitting exponential curves to the data. Red lines represent the mean ± 95% confidence intervals. For comparison of growth rates, P- values were determined using the Kolmogorov–Smirnov non-parametric test. Full size image When M. tuberculosis was exposed to 10-fold lower BDQ (30 × MIC) significant lysis (46%) was observed, but interestingly some of the cells continued to elongate in presence of the drug ( Supplementary Fig. 2 , Supplementary Movie 2 ). This suggests that either the intracellular concentrations of BDQ in these bacteria were not sufficient to completely shut down ATP synthesis or that these bacteria were able to generate enough ATP using alternate mechanisms to extend their survival. Global transcriptional response of M. tuberculosis to BDQ Insight into the changes in bacterial energy metabolism that assist in survival under conditions of ATP depletion may provide clues for the delayed onset of bacterial killing. We examined the global transcriptional response of mycobacteria to BDQ, focusing on the changes in the gene expression profile during the initial phase of treatment (30, 180 and 360 min) ( Fig. 3a ). Genes showing the strongest upregulation at 30 and 180 min time points belong to the mycobacterial dormancy regulon ( Fig. 3a , tables below panels). We observed a transient induction of all 39 genes of the dormancy regulon represented in our microarray analysis at 30 and 180 min, whereas at 360 min the expression profile of this regulon largely resembled the baseline profile (0 min) ( Fig. 3b ). This so-called dormancy regulon is a set of 48 genes that are induced when M. tuberculosis responds to multiple stresses, including the transition between respiring and nonrespiring conditions, redox stress or poisoning by nitric oxide [20] , [21] , [22] , [23] . The dormancy regulon has been associated with metabolic states requiring less ATP and is postulated to play a role in sustaining bacterial ATP levels [19] , [23] , [24] . The upregulation of the dormancy regulon observed here in response to BDQ may act as a bacterial defence mechanism to countract cellular ATP depletion and may thus contribute to the temporal delay in bacterial killing. 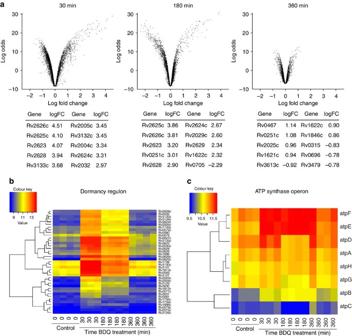Figure 3: Transcriptional response ofM. tuberculosisto BDQ treatment. (a) Global gene expression changes 30, 180 and 360 min after addition of BDQ (30 × MIC). The volcano plot shows the log2-fold changes in gene expression induced by BDQ as compared with untreated control. The log odds describe the probability that the gene indeed is differentially expressed, a zero value corresponds to a 50-50 chance of differential expression. Genes were ranked based on their absolute log2-fold change and the 10 genes with highest differential regulation at each time point (dots highlighted in red in the volcano plots) are listed below the respective panels. For all listed genes differential regulation was significant (P<0.05, determined using the moderatedt-statistics). A list of top 20 regulated genes is presented inSupplementary Data 1. (b,c) Expression of the dormancy regulon (b) and the ATP synthase operon (c) at 30, 180 and 360 min of BDQ treatment. The colour scales represent log2-fold changes in gene expression. Figure 3: Transcriptional response of M. tuberculosis to BDQ treatment. ( a ) Global gene expression changes 30, 180 and 360 min after addition of BDQ (30 × MIC). The volcano plot shows the log 2 -fold changes in gene expression induced by BDQ as compared with untreated control. The log odds describe the probability that the gene indeed is differentially expressed, a zero value corresponds to a 50-50 chance of differential expression. Genes were ranked based on their absolute log 2 -fold change and the 10 genes with highest differential regulation at each time point (dots highlighted in red in the volcano plots) are listed below the respective panels. For all listed genes differential regulation was significant ( P <0.05, determined using the moderated t -statistics). A list of top 20 regulated genes is presented in Supplementary Data 1 . ( b , c ) Expression of the dormancy regulon ( b ) and the ATP synthase operon ( c ) at 30, 180 and 360 min of BDQ treatment. The colour scales represent log 2 -fold changes in gene expression. Full size image Transcriptomic data also revealed that genes belonging to the ATP synthase operon are upregulated ( Fig. 3c ), presumably initiated by feedback mechanisms triggered by depletion of cellular ATP levels. This upregulation probably reflects a strategy to counteract the inhibition of ATP synthase during the initial phases of BDQ exposure. Upregulation of representative components of both the dormancy regulon and the ATP synthase operon was confirmed by quantitative reverse transcriptase real-time polymerase chain reaction ( Supplementary Fig. 3a,b ). Apart from the strong induction of dormancy and ATP synthase genetic components seen at 30 min and 180 min time points, transcriptome data at 360 min time point revealed moderate upregulation of the isocitrate lyase ( rv0467 ) and of the cytochrome bd complex ( rv1621c , rv1622c , rv1623c ), in addition to proteins of hypothetical function ( Fig. 3a ). Both isocitrate lyase, a key enzyme of the glyoxylate pathway, and cytochrome bd, an alternative electron acceptor in the respiratory chain, are prominent components of energy metabolic pathways under conditions of physiological stress, such as during mouse lung infection, in human macrophages or in the presence of inhibitors of energy metabolism [25] , [26] , [27] . In contrast, pronounced downregulation was observed for two components of the large ribosomal subunit ( rv0703 and rv0719 , 180 min) ( Supplementary Data 1 ). This suggests downregulation of protein synthesis thereby limiting cellular ATP consumption. Proteomic response of M. tuberculosis to BDQ Coupled to our understanding of the global transcription profile, we performed quantitative protein analysis on M. tuberculosis treated with BDQ. Using a mass spectrometric approach with isobaric tagging for relative quantification (iTRAQ)-labelling we identified a total of >1,500 proteins and determined their differential expression 6 and 24 h after BDQ exposure (10 × MIC) (detailed in Supplementary Data 2–4 ). For a global overview of key changes in metabolism upon BDQ exposure proteins displaying high differential regulation (top 100 proteins at each time point) were grouped into functional categories based on the TubercuList server classification [28] . At both 6 and 24 h time points, BDQ treatment most prominently affected intermediate metabolism and respiration ( Fig. 4a ), reflecting the drug’s unique mechanism of action. Prominent differential regulation was also observed for proteins involved in cell wall and cell processes, information pathways and lipid metabolism as well as for conserved hypothetical proteins ( Fig. 4a ). 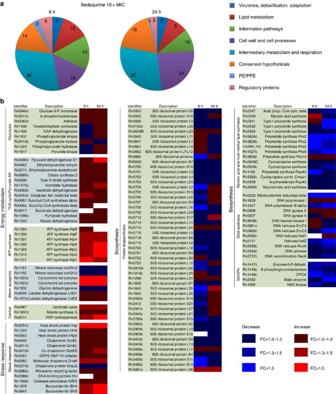Figure 4: Proteomic response ofM. tuberculosisto BDQ treatment. (a) Global proteome response and contribution of different metabolic categories. Proteins displaying the highest differential regulation factors (top 100 proteins) 6 or 24 h after addition of BDQ (10 × MIC) were grouped according to the TubercuList classification. (b) Heat map representing differential regulation of biochemical pathways related to energy metabolism (left row) or to biosynthetic pathways (middle row and right row). The colour scale indicates differential regulation as the FC of protein amount relative to untreated control. Upregulation is indicated in red, downregulation in blue. For a complete overview of detected and identified proteins please refer toSupplementary Data 2; detected peptides are presented inSupplementary Data 3 and 4. Figure 4: Proteomic response of M. tuberculosis to BDQ treatment. ( a ) Global proteome response and contribution of different metabolic categories. Proteins displaying the highest differential regulation factors (top 100 proteins) 6 or 24 h after addition of BDQ (10 × MIC) were grouped according to the TubercuList classification. ( b ) Heat map representing differential regulation of biochemical pathways related to energy metabolism (left row) or to biosynthetic pathways (middle row and right row). The colour scale indicates differential regulation as the FC of protein amount relative to untreated control. Upregulation is indicated in red, downregulation in blue. For a complete overview of detected and identified proteins please refer to Supplementary Data 2 ; detected peptides are presented in Supplementary Data 3 and 4 . Full size image On the basis of these top-line findings, we subsequently focused on metabolic pathways connected to synthesis or consumption of cellular ATP. Proteins belonging to these metabolic pathways were selected and their differential regulation was presented in a heat map ( Fig. 4b ). We regarded proteins showing an increase or decrease with a fold change (FC)>1.5 as strongly regulated, those with fold change 1.3<FC<1.5 as moderately regulated and proteins with fold change 1.0<FC<1.3 as not regulated. Components of the ATP synthase complex were induced, with strong upregulation found for one subunit at 6 h and for three subunits at 24 h time point ( Fig. 4b , left panel), reflecting a strategy to compensate for inhibition of ATP synthesis. Enzymes of the glycolytic pathway did not display differential regulation ( Fig. 4b , left panel). Two components of the tricarboxylic acid cycle, 2-oxoglutarate ferredoxin oxidoreductase subunit β and aconitate hydratase, were moderately upregulated at 6 and 24 h time point, respectively ( Fig. 4b , left panel). Moreover, the PdhB subunit of the pyruvate dehydrogenase complex, an enzyme linking glycolysis with the tricarboxylic acid cycle, was strongly upregulated at 24 h of treatment ( Fig. 4b , left panel). Unlike the typical mycobacterial response to growth arrest, where the tricarboxylic acid cycle is considerably downregulated [29] , this central metabolic pathway apparently remains functional during bacteriostasis triggered by BDQ. Activity of this central cycle may help to evade BDQ-induced antibiotic stress by providing precursors for certain essential biosynthetic processes or by modulating pressure on the respiratory chain. The observed usage of alternative electron acceptors such as cytochrome bd, which was strongly upregulated at both time points ( Fig. 4b , left panel), may assist in maintaining the respiratory electron flow. Induction of isocitrate lyase and of phosphoenolpyruvate-carboxykinase indicates a re-routing of central carbon metabolism in response to BDQ exposure ( Fig. 4b , left panel), which is reminiscent of the redistribution of carbon flow reported for M. tuberculosis upon lung infection [29] . Two components of the stress response, the heat shock protein Rv0251c and bacterioferritin, were strongly upregulated (Rv0251c at 6 and 24 h time points, bacterioferritin at 24 h time point) ( Fig. 4b , left panel). Induction was also observed for various other components of the stress response, for example, moderate upregulation was found for the co-chaperonin GroES after 24 h of treatment and for the DnaK protein at both 6 and 24 h time point ( Fig. 4b , left panel). Induction of these facilitators of protein (re-)folding may contribute towards optimizing the integrity of synthesized proteins or to recycling of existing proteins. In contrast, major biosynthetic pathways were generally found downregulated upon BDQ treatment, including ribosomal protein synthesis, DNA biosynthesis and synthesis of mycolic acids, a key component of the mycobacterial cell envelope [30] ( Fig. 4b , right panel). Strong downregulation was observed for several polyketide synthases, several ribosomal subunits and for DNA helicase and a ribonucleotide-diphosphate reductase subunit, which are components of lipid, protein and DNA biosynthesis, respectively ( Fig. 4b , right panel). This suggests that in response to ATP depletion via inhibition of ATP synthase by BDQ bacteria try to evade shortage of energy by minimal usage of ATP consuming processes. To support this observation, we measured protein and DNA synthesis activity in mycobacteria grown in presence of BDQ ( Supplementary Fig. 4 ). BDQ blocked both protein and DNA synthesis in a dose-dependent manner, in line with the our proteome data. Taken together, the observed changes in the mycobacterial proteome reflect a general strategy employed by mycobacteria for preserving ATP pools, minimizing consumption of cellular ATP and enhancing the capacity of ATP-generating pathways. Influence of BDQ on bacterial NADH/NAD + redox balance In addition to changes occurring in the transcriptome and proteome of M. tuberculosis we also assessed the impact of the drug on bacterial redox balance. We determined the intracellular ratio of NADH, a central redox cofactor of the bacterial cell, versus its reduced version NAD + during the initial period of BDQ exposure. BDQ at 3 or 30 × MIC caused elevated cellular NADH/NAD + ratios within 24 h after drug addition ( Fig. 5a ), indicating that the intracellular NADH/NAD + redox balance is shifted towards a reducing state. This change may be due to blockage of ATP synthase by BDQ, which likely exerts back pressure on the mycobacterial respiratory chain, thereby impeding the respiratory electron flow and in turn diminishing rates of NADH oxidation. Disturbed NADH/NAD + redox balance may trigger activation of the dormancy regulon via reduction of its DosS sensor kinase [31] , [32] , thereby assisting in adaptation to BDQ-induced stress. 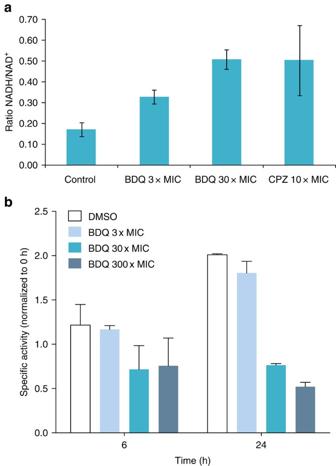Figure 5: BDQ and bacterial redox balance. (a) Cellular NADH/NAD+ratios in mycobacteria treated with BDQ.M. tuberculosiswas grown in 7H9 medium in the presence of the indicated concentrations of BDQ. 24 h after BDQ addition cell extracts were prepared using a French Press and the NADH and NAD+concentrations were measured using yeast alcohol dehydrogenase. Two independent experiments were done, one of them in duplicate. Mean values and s.e.m. are shown. (b) Glyceraldehyde-3-phosphate dehydrogenase activity in mycobacteria treated with BDQ.M. tuberculosiswas grown in 7H9 medium with the indicated concentrations of BDQ to an OD=0.8–1.0. Cell extracts were prepared using bead-beating in a homogenizer. The reaction rate was measured by monitoring the absorption of produced NADH at 340 nm. Specific enzyme activity (μmol min−1mg−1) was normalized to the 0 h time point and plotted. Data shown are the mean+s.e. of two independent experiments. Figure 5: BDQ and bacterial redox balance. ( a ) Cellular NADH/NAD + ratios in mycobacteria treated with BDQ. M. tuberculosis was grown in 7H9 medium in the presence of the indicated concentrations of BDQ. 24 h after BDQ addition cell extracts were prepared using a French Press and the NADH and NAD + concentrations were measured using yeast alcohol dehydrogenase. Two independent experiments were done, one of them in duplicate. Mean values and s.e.m. are shown. ( b ) Glyceraldehyde-3-phosphate dehydrogenase activity in mycobacteria treated with BDQ. M. tuberculosis was grown in 7H9 medium with the indicated concentrations of BDQ to an OD=0.8–1.0. Cell extracts were prepared using bead-beating in a homogenizer. The reaction rate was measured by monitoring the absorption of produced NADH at 340 nm. Specific enzyme activity (μmol min −1 mg −1 ) was normalized to the 0 h time point and plotted. Data shown are the mean+s.e. of two independent experiments. Full size image On the other hand, elevated NADH/NAD + ratios disturb cellular redox balance and may concomitantly inhibit metabolic pathways involved in production of NADH. To validate this observation, we measured the activity of glyceraldehyde-3-phosphate dehydrogenase, a central enzyme in the glycolytic pathway, in a biochemical assay. We found significantly lower activity after 24 h of BDQ treatment as compared with untreated controls ( Fig. 5b ). Impact of energy source for drug susceptibility On the basis of the proteome results indicating functional glycolyic pathways and tricarboxylic acid cycle during the initial phase of BDQ treatment, we explored the impact of the employed energy source on killing of M. tuberculosis by BDQ. Fermentable energy sources such as glycerol or glucose allow for ATP synthesis by glycolysis or by oxidative phosphorylation using ATP synthase. With fatty acids as energy source, the bacteria cannot utilize the glycolytic pathway and ATP production is restricted to oxidative phosphorylation with ATP synthase. For these reasons mycobacteria using fatty acids as energy source may display enhanced susceptibility to BDQ. As depicted in Fig. 6 , M. tuberculosis grown on fatty acids, such as oleic acid, propionic acid or sodium acetate, displayed accelerated killing by BDQ within the initial days of treatment as compared with controls grown on glycerol or glucose. In particular bacteria grown in presence of oleic acid as energy source yielded enhanced bacterial susceptibility to BDQ exposure as compared with glycerol as the standard medium ( P <0.05 on 5 of the 7 initial days, determined by t -test). For propionic acid and sodium acetate the enhancement of killing was less pronounced ( P <0.05 on two days and on one day, respectively). This finding has important implications since it has been proposed that the mycobacterial sub-population residing in human macrophages primarily utilizes fatty acids as energy source [27] , [33] . Our results may therefore in part explain the strong bactericidal activity observed for BDQ in mycobacteria-infected macrophages, where the intracellular potency of BDQ exceeded its extracellular activity [16] . Interestingly, for the front-line anti-TB drugs the killing of M. tuberculosis in lipid-loaded macrophages was found to be significantly reduced [34] . Thus, inhibitors of respiratory ATP synthesis may be particularly suitable for the eradication of this difficult to kill minority sub-population of M. tuberculosis in the human host cells. 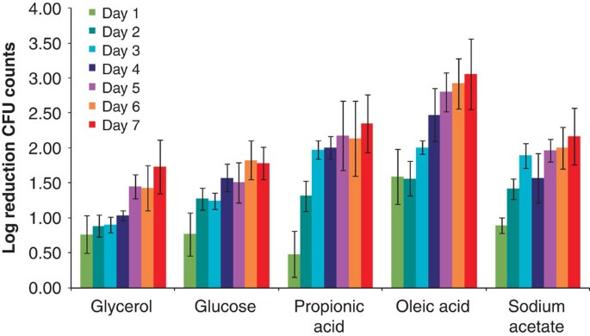Figure 6: Influence of the supplemented energy source on killing ofM. tuberculosisby BDQ. 7-day kill kinetics were measured forM. tuberuclosisin liquid culture (7H9 medium) supplemented with the indicated energy sources in the presence of BDQ (30 × MIC). The experiments were done three times; mean values and s.e.m. are shown. Figure 6: Influence of the supplemented energy source on killing of M. tuberculosis by BDQ. 7-day kill kinetics were measured for M. tuberuclosis in liquid culture (7H9 medium) supplemented with the indicated energy sources in the presence of BDQ (30 × MIC). The experiments were done three times; mean values and s.e.m. are shown. Full size image Our findings suggest that exposure of M. tuberculosis to BDQ triggers metabolic remodelling to counteract ATP depletion. Bacterial killing is associated with depletion of cellular ATP by more than 10-fold. In the intial phase of BDQ-induced bacteriostasis, remodelling of ATP consuming and ATP producing pathways may enable maintenance of ATP levels sufficient for bacterial viability for several days and concomitantly prevent killing. Utilization of the glycolytic pathway may contribute sufficient ATP for short-term survival, but on continued inhibition of ATP synthase, this alternative pathway apparently is not sufficient. It can be speculated that increased cellular NADH/NAD + ratios cause a decrease in glycolytic rates, thereby preventing adequate ATP production by glycolysis. In this regard, factors linking cellular ATP depletion with bacterial death need to be elucidated to shed light on bacterial killing by inhibitors of energy metabolism in particular and on the mechanism of killing by bactericidal antibiotics in general. It is important to understand if the metabolic response to BDQ is a non-specific defence mechanism or is more specific to this antibacterial drug. Cessation of growth, decreased cellular ATP levels, upregulation of the dormancy regulon as well as downregulation of protein and DNA biosynthesis pathways has been reported for mycobacteria during dormancy [19] , [20] , [24] , [35] , adaptation to the macrophage environment [25] or upon mouse lung infection [29] , [36] . However, BDQ induces a distinct response in terms of upregulation of energy metabolic pathways, particularly the ATP synthase, which is not observed under conditions of general stress or bacteriostasis [29] , [36] , [37] . Stimulation of the dormancy regulon, observed here upon inhibition of ATP synthase by BDQ, apparently does not represent a general response to inhibition of energy metabolism, as several inhibitors of respiratory functions, such as chlorpromazine or potassium cyanide, did not cause significant induction of the dormancy response [26] . In contrast, increased cytochrome bd expression, as found here in the presence of BDQ, was previously reported in response to a broad range of inhibitors of energy metabolism and in related metabolic stress situtations [26] , [36] , [38] , reflecting a more general role of the cytochrome bd in the transition between bacterial (energy) metabolic states. The link between inhibition of ATP synthase by BDQ and the subsequent induction of the dormancy regulon may be due to multiple factors, like decreasing cellular ATP levels or changes in intracellular redox state. Decreasing ATP levels may via unknown cellular ATP sensors activate the dormancy regulon. ATP sensors have been reported for several bacterial species [39] , [40] , [41] and it can be speculated that ATP sensing factors, such as members of the univeral stress protein family [42] , may be involved in the mycobacterial response to external stresses influencing bacterial ATP levels. Alternatively, a reduced state of the bacterial respiratory chain, as indicated by the elevated NADH/NAD + ratios, may activate the DosS sensor kinase, which has been reported to be a redox sensor [31] , [32] . BDQ-triggered induction of the dormancy regulon is transient with gene expression essentially returning to baseline level after 6 h. This period is shorter as compared with dormancy regulon induction by nitric oxide [20] ; however, a transient nature of dormancy regulon induction with the majority of genes returning to baseline levels has been reported previously for M. tuberculosis in a defined hypoxia model [38] . The duration of dormancy regulon induction and the level of gene expresion in the new steady state may significantly depend on the type of stress applied or on the model system used. In this regard, defining the bacterial regulatory network related to BDQ-induced metabolic changes, as recently reported for M. tuberculosis in response to hypoxia and re-aeration [43] , may assist in pinpointing key nodes of metabolic interactions linked to induction and cessation of the dormancy response. For new anti-TB drug candidates targeting energy metabolic pathways using eBA as an efficiency surrogate may underestimate their clinical potency. Apart from BDQ, delayed bactericidal activity has also been reported for other investigational drugs, such as PA-824 and delamanid, which likely inhibit multiple targets including respiratory chain cytochrome oxidases [13] , [44] . The recently discovered drug Q203, which targets the cytochrome bc 1 complex of the mycobacterial respiratory chain, was also slow acting during the first 2 weeks of treatment in a mouse model of acute tuberculosis infection [45] . This might suggest a general phenomenon of delayed onset of bactericidal activity for respiratory inhibitors, including clofazimine that also targets respiratory chain, which might be due to metabolic remodelling as revealed here for BDQ. Certain pharmacological and clinical factors, such as time to steady state, protein binding and distribution into fibrotic lesions, cavities and granulomas may affect the effective drug concentrations at the target sites and also influence a drug’s initial activity. The efficacy of drug candidates targeting respiratory ATP synthesis may be underestimated in in vitro studies employing standard growth media [46] , [47] , which contain glycerol and glucose as the primary energy sources. The strong bactericidal effect of BDQ towards bacteria grown on lipids suggests that for microbiological characterization of new inhibitors targeting respiratory ATP synthesis fatty acids or related non-fermentable energy sources might be explored. In addition, these results highlight the importance of energy metabolism inhibitors in combating mycobacteria residing in lipid-rich micro-environments. As such, new drug candidates targeting ATP synthase and associated metabolic processes are expected to have potent activity in humans. Kill kinetics on M. tuberculosis M. tuberculosis H37Rv was cultured in 7H9 broth to mid-log phase. Bacteria were diluted to ~10 6 CFU ml −1 . BDQ was added at 0.1, 1 and 10 μg ml −1 , isoniazid at 10 μg ml −1 . At indicated time points, samples were taken and CFU counts were performed. Cellular ATP level measurement of M. tuberculosis M. tuberculosis H37Rv was cultured in 7H9 broth to mid-log phase. Bacteria were diluted to ~10 6 CFU ml −1 . BDQ was added at 0.1, 1 and 10 μg ml −1 , isoniazid at 10 μg ml −1 . At indicated time points, samples were taken, and 1.5 ml bacteria suspension was mixed with 3 ml boiling Tris-EDTA reagent (100 mM Tris, 4 mM EDTA, pH 7.75) and mixed for 2 min with glass beads, heated at 100 °C for 5 min and cooled on ice. Cell debris was removed by centrifugation. An equal volume of luciferase reagent (ATP Bioluminescence Assay Kit HS II, Roche) was added to the supernatant and luminescence was measured. The majority of bacteria at day 18 were not lysed as determined by microscopy ( Fig. 2 ) but could not be counted on plates ( Fig. 1a ). For this reason, ATP levels were expressed per ml of culture [23] and not per CFU. Impact of energy source on efficacy of BDQ on M. tuberculosis M. tuberculosis H37Rv was cultured in 7H9 broth to mid-log phase. Bacteria were diluted to ~10 6 CFU ml −1 in Middlebrook 7H9 medium or in Middlebrook medium with, respectively, 2% glucose, 0.1% propionic acid, 0.01% oleic acid or 0.1% sodium acetate. Bacteria were adapted to the new media for 24 h. BDQ was added at 1 μg ml −1 , isoniazid at 10 μg ml −1 . Kill kinetics and cellular ATP levels were performed daily for 7 days. Time-lapse imaging For purposes of imaging, M. tuberculosis expressing GFP was constructed by transforming with the attB-integrating vector pND235 (Wakamoto et al. [48] ). Cells were grown in 7H9 medium at 37 °C to mid-log phase and were seeded into a custom-made microfluidic device as described before [48] . Briefly, bacteria from mid-exponential cultures were concentrated 10-fold by centrifugation and were passed through a 5 μm filter (Millipore) to get rid of clumps. 2 μl of these filtered bacteria were sandwiched between the coverslip and a cellulose membrane, on top of which the microfluidic device was placed. This whole assembly was secured in a custom-built acrylic frame and placed on the microscope stage for imaging [48] . The inlet tube connected to the microfluidic device was connected to a syringe containing fresh 7H9 medium and the outlet tubing was directed to the waste receptacle. Medium (with or without drug) was replaced every 20 h. Medium was pumped through the syringe pump at a flow rate of 25 μl min −1 . Images were acquired at 1 h intervals on the phase and FITC (excitation 490/20; emission 528/38) channels using a DeltaVision personalDV imaging system (Applied Precision) equipped with a × 100 objective (Olympus UPLFL 100X PH, 1.3 NA) and a CoolSnap HQ2 camera. As an end point assay, 1.0 μg ml −1 propidium iodide was added to the flow medium for 24 h to stain cells with permeabilized cell envelopes and imaging done on the red channel (excitation 555/28; emission 617/73). Analysis of the time-lapse image stacks was carried out using ImageJ v 1.47a ( http://rsb.info.nih.gov/ij/ ). Area of individual cells was measured using the polygon function and single-cell growth rates were calculated by fitting the curves with exponential growth function. The survival curves depicted in Supplementary Fig. 1 and Supplementary Fig. 2 were generated by tracking cell division and lysis events over the course of the experiment using the ‘Cell Counter’ plugin of ImageJ. Cytolysis was scored visually by abrupt loss of GFP fluorescence and abrupt decrease in phase intensity. Statistic analysis and fitting of data was performed using Prism (GraphPad). For comparison of growth rates, P- values were determined using the Kolmogorov–Smirnov non-parametric test. Transcriptome analysis For RNA isolation, M. tuberculosis H37Rv was cultured in 7H9 broth to mid-log phase. BDQ was added at final concentration of 1 μM. At 0.5, 1, 3 and 6 h after addition of the compound, 10 ml of culture was pelleted and resuspended in 1 ml of RNAprotect Bacteria Reagent. Bacteria were pelleted again, resuspended in RLT-buffer with β-mercaptoethanol and mechanically disrupted with Mixer Mill MM 310. Only the supernatant was used for RNA extraction using RNeasy Protect Bacteria Mini kit (Qiagen). RNA was eluted in RNAse free water. Four biological replicates were used to extract RNA from M. tuberculosis cultures. For the 1 h time point the RNA quality and RNA yield was affected, possibly due to effects of the compound on the bacteria. As the resulting array data for the 1 h time point were inconclusive, they were not taken into consideration for the interpretation, but included in the data submission to the GEO repository. For labelled cDNA preparation, reverse transcription was performed on 5 μg of total RNA using random primers and Superscript II RT (Invitrogen Life Technologies). For the reaction, 750 ng random hexamers were mixed with the RNA in a total volume of 30 μl and heated to 70 °C for 10 min. After cooling to 25 °C for 10 min, the first strand reagents were added and incubated for 1 h at 37 °C followed by 1 h at 42 °C. SuperScript II was heat inactivated at 70 °C for 15 min and the mixture cooled to 4 °C. The template RNA was removed using RNase H (Invitrogen) and RNase A/T1 cocktail (Ambion) at 37 °C for 20 min in 100 μl total volume. The cDNA was purified using the QiaQuick PCR purification kit from Qiagen. The purified cDNA was than fragmented using DNAse I in 1 × One-Phor-All buffer (GE Healthcare) for 20 min. If the bulk of DNA was not at 50–100 bp, the digest was repeated. After fragmentation a 3′-end terminal labelling was performed for 2 h at 37 °C using the BioArray Terminal Labeling Kit with Biotin-ddUTP, (ENZO Diagnostics, Farmingdale, NY P/N 900181). The fragmented and end-labelled cDNA was added to the hybridization solution. For microarray analysis, samples were processed on TB_ALL GeneChips with antisense probes (Affymetrix, Santa Clara, CA, part # 510285) containing ~6,000 probe sets interrogating 3,924 ORFs and 738 intergenic regions of M. tuberculosis H37Rv. For hybridization, staining and scanning the Affymetrix E. coli Antisense Genome Array protocol was followed. Hybridization was performed for 18 h at 45 °C under continuous rotation according to the recommendations of Affymetrix. Arrays were stained in Affymetrix Fluidics stations using Streptavidin/Phycoerythrin followed by staining with anti-streptavidin antibody and a second Streptavidin/Phycoerythrin staining. Subsequently, arrays were scanned with a Genechip scanner. All data analysis was done in R (version 2.14.1) using BioConductor packages (version 2.9). Data preprocessing was done with no background correction, vsn normalization and summarization using median polish. Differential gene expression was calculated using the BioConductor package limma [49] ( http://www.bioconductor.org/packages/release/bioc/vignettes/limma/inst/doc/usersguide.pdf ), with default settings. Log odd values were automatically adjusted for multiple testing. For reverse transcription quantitative PCR, first strand cDNA synthesis was performed on 0.5 μg total RNA using random hexamer primers and Superscript II RT (Invitrogen Life Technologies). TaqMan FAM and TAMRA probes (Eurogentec) and primers for the mycobacterial genes were designed using the Primer Express software (version 2.0.0, Applied Biosystems); a list of primers provided as Supplementary Table 1 . Amplification of endogenous 16S ribosomal RNA was performed to standardize the amount of cDNA sample added to each reaction. Real-time quantification was carried out using the ABI PRISM 7900HT Sequence Detection System (Applied Biosystems) as described by the manufacturer. Serial dilutions of various cDNAs were used to generate standard curves of threshold cycles versus the logarithms of concentration for 16S ribosomal RNA and the genes of interest. A linear regression line calculated from the standard curves allowed determination of transcript levels in the RNA samples by the relative quantification method. Proteome analysis For sample collection, M. tuberculosis H37Rv was cultured in 7H9 broth to mid-log phase. BDQ was added at final concentration of 1 and 10 × MIC and isoniazid at 1 × MIC. After 6 and 24 h after addition of the compound, 50 ml of culture (one biological replicate) was washed with PBS and pelleted. Bacteria were heat-killed and resuspended in 2 ml lysis buffer (8.9 M urea, 2% Triton X-100, 2% IPG-buffer (Roche), 0.13 M DTT, 8 mM PMSF). The lysate was passed three times through the French Press at 14,000 Psi in a small cell. Cell debris was removed by centrifugation and supernatant was collected. For protein digestion, the proteins were cleaned up from the cell lysis buffer by cold ethanol/acetone precipitation. The pellets were resuspended in 6 M urea, 2 M thiourea, 50 mM triethyl ammonium bicarbonate (TEAB), pH 8.0. The proteins were reduced with 20 mM dithiothreitol for 1 h at 30 °C followed by alkylation with 50 mM iodoacetamide for 30 min in the dark. The samples were diluted 1:8 with 50 mM TEAB, pH 8.0 and digested with trypsin over night at room temperature. After digestion the samples were acidified to a final concentration of 2% formic acid and centrifuged at 12,000 g for 10 min to precipitate the lipids. Before iTRAQ labelling, the supernatants were desalted and dried down using vacuum centrifugation. For iTRAQ labelling, the peptides were resuspended in 200 mM TEAB, pH 8.0. A total of 100 μg for M. tuberculosis H37Rv and 50 μg for the other conditions were labelled (H37Rv BDQ 1 × MIC 6+24 h; H37Rv BDQ 10 × MIC 6+24 h and H37Rv isoniazid 1 × MIC 6+24 h) with 4-plex iTRAQ (Applied Biosystems, Foster City, CA). The labelling was performed as described by the manufacturer. After labelling, the samples were mixed 1:1:1:1 and dried down using vacuum centrifugation. For nano-LC MS/MS, the peptide mixtures were fractionated by loading 20 μg samples on a HPLC Agilent 1200 system with a homemade TSKGel Amide-80 HILIC column. The peptides were eluted with an inverse gradient from 100% B (90% ACN; 0.1% TFA) to 60% B in 30 min with an increasing amount of A-solvent (0.1% TFA). The HILIC fractions were further analysed by an EASY nano-HPLC system (Thermo Fischer Scientific) connected to an LTQ OrbiTrap XL mass spectrometer (Thermo Fisher Scientific). The nano-HPLC system was equipped with a self-packed 15-cm analytical column (100 μm ID, 360 μm OD, ReproSil-Pur C18 AQ 3 μm; Dr Maisch, Germany). The mass spectrometer was operated in positive ion mode and a data-dependent acquisition method that automatically switched between MS and MS/MS was employed. The most three intense ions from the MS spectra were fragmented by collision induced dissociation in the LTQ and additionally fragmented by high-energy collision induced dissociation (HCD) with detection in the OrbiTrap analyser. The HCD fragmentation is necessary to obtain abundant iTRAQ reporter ions for later quantitation. The raw MS/MS data were analysed using Proteome Discoverer v1.3 beta (Thermo Scientific). MS/MS spectra were converted to .mgf files and searched against the NCBI database (taxonomy: Mycobacterium tuberculosis H37Rv). Database search was performed with the following fixed parameters: precursor mass tolerance 10 p.p.m. ; MS/MS mass tolerance 0.8 Da for collision induced dissociation data or 0.05 Da for HCD data and trypsin as protease with up to two missed cleavages. Variable modifications included: methionine oxidation and N-terminal and lysine 4-plex iTRAQ label. A concatenated decoy database search was performed, which was derived from the NCBI M . tuberculosis H37Rv database. Peptides with a FDR of 5% and an ion score of 20 (MudPit scoring) and Rank 1 were accepted. Protein identifications were accepted when minimum two peptides/protein were identified and the protein had a score of 30 or higher. iTRAQ quantification was performed using Proteome Discoverer with reporter ion integration within a 50 p.p.m. window. The quantification was based on a relative quantification, means the intensities from the reporter ions from every condition (wild type H37Rv BDQ 1 × MIC 6+24 h; wild type H37Rv BDQ 10 × MIC 6+24 h and wild type H37Rv isoniazid 1 × MIC 6+24 h) were compared with the intensity of the reporter ion of the wild type H37Rv (control). The intensities of the reporter ion from the certain conditions were divided by the reporter ion intensity from the wild type H37Rv to obtain a peptide ratio for every identified peptide. The protein ratios were than calculated based on the peptide ratios of the individual proteins. The peptide ratios were log 2 transformed and normalized against the median. The protein ratios (fold change) were than calculated based on the peptide ratios of the individual proteins. Strongly regulated proteins were determined based on the 1.5-fold change and moderately regulated proteins with a 1.3-fold change, a cutoff often chosen for biological significance [50] . Glyceraldehyde-3-phosphate dehydrogenase assay M. tuberculosis was cultured in 7H9 broth and grown to an A 600 nm of 0.8. Cultures were treated with 0.1, 1 or 10 μg ml −1 BDQ for 6 and 24 h. Control cultures were treated with dimethylsulphoxide. Culture aliquots (10 ml) were harvested and resuspended in cell lysis buffer—50 mM Tris pH 8.0, 10% glycerol, containing protease inhibitor cocktail (Roche, Switzerland). Cell lysis was carried out by bead-beating using 0.1 mm zirconia beads in a Precellys-24 homogenizer (Biolabo, Switzerland). Glyceraldehyde-3-phosphate dehydrogenase activity was measured in whole cell protein extracts by following NADH formation measuring absorbance at 340 nm, as per the procedure described previously [51] . Assay was performed at 37 °C in 200 μl of assay buffer comprising 0.015 M sodium pyrophosphate buffer pH 8.5, 0.03 M sodium arsenate, 2.5 mM NAD + , 2.5 mM glyceraldehyde-3-phosphate. The assay mixture (without the substrate) was mixed with 10 μg of protein extract and shaken at 37 °C to equilibrate the temperature. The reaction was initiated by addition of the substrate, glyceraldehyde-3-phosphate. Controls included wells without protein extract or without the substrate. Purified NADH (Sigma) was used to generate calibration curves. One unit is defined as the quantity of enzyme reducing 1 μmol NAD + min −1 mg −1 of protein extract. NADH/NAD + assay M. tuberculosis was cultured in 7H9 broth and grown to an A 600 nm of 0.8. Cultures were treated with 0.1, 1 or 10 μg ml −1 BDQ for 24 h. NADH and NAD + concentrations were determined and the NADH/NAD + ratio was calculated as described [52] . Briefly, bacteria were harvested, resuspended in 0.2 M HCl (for NAD + extraction) or in 0.2 M NaOH (for NADH extraction), heated at 55 °C for 10 min and cooled on ice. Cell debris was removed by centrifugation. The supernatant was preincubated for 5 min in the dark in Bicine buffer containing EDTA, ethanol, 3-[4,5-dimethylthiazol-2-yl]-2,5-diphenyltetrazolium bromide (MTT), and phenazine ethosulfate. The reaction was started by addition of yeast alcohol dehydrogenase II and the absorbance at 570 nm was recorded for 10 min. Accession codes: Microarray data have been deposited in the GEO repository under accession code GSE43749 . How to cite this article: Koul, A. et al. Delayed bactericidal response of Mycobacterium tuberculosis to bedaquiline involves remodelling of bacterial metabolism. Nat. Commun. 5:3369 doi: 10.1038/ncomms4369 (2014).